A microscopic view on the Mott transition in chromium-doped V2O3 V 2 O 3 is the prototype system for the Mott transition, one of the most fundamental phenomena of electronic correlation. Temperature, doping or pressure induce a metal-to-insulator transition (MIT) between a paramagnetic metal (PM) and a paramagnetic insulator. This or related MITs have a high technological potential, among others, for intelligent windows and field effect transistors. However the spatial scale on which such transitions develop is not known in spite of their importance for research and applications. Here we unveil for the first time the MIT in Cr-doped V 2 O 3 with submicron lateral resolution: with decreasing temperature, microscopic domains become metallic and coexist with an insulating background. This explains why the associated PM phase is actually a poor metal. The phase separation can be associated with a thermodynamic instability near the transition. This instability is reduced by pressure, that promotes a genuine Mott transition to an eventually homogeneous metallic state. Hitherto, the phase diagram of V 2 O 3 (see Fig. 1a ) was mainly established by means of transport measurements, that is detecting the electronic response on a macroscopic spatial scale [1] . According to this phase diagram, V 2 O 3 exhibits a first-order MIT from a low-T antiferromagnetic insulating state (AFI) to a paramagnetic metallic state (PM) when T exceeds T N ~160 K. A different, paramagnetic insulating state (PI) is reached at T > T N if V is partially substituted by Cr. Within a narrow range of Cr content (0.005< x <0.018) a PI to PM transition is obtained on reducing the temperature across a T MIT > T N with a slight discontinuity of the lattice parameters within the same corundum phase. In particular (V 0.989 Cr 0.011 ) 2 O 3 has attracted great interest since its discovery in 1969 [1] , because it provides the opportunity to span all phases, through two MITs. One (AFI↔PM) shows both a change of crystal symmetry and of magnetic state, the other (PM↔PI) is iso-structural and a prototype of the correlation-driven Mott transition. 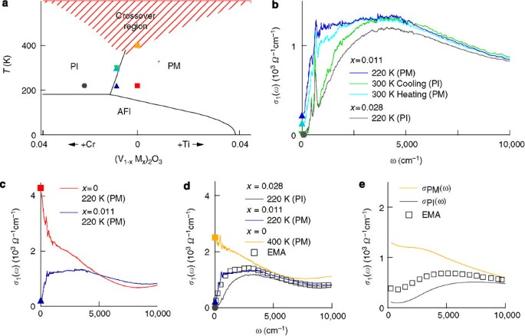Figure 1: Temperature-dependent infrared measurements. (a) Schematic phase diagram as defined in (ref.1); markers indicate the measurements shown in (b–e) in the same colour coding. (b)σ1(ω) of (V1−xCrx)2O3forx=0.011 and 0.028 at selectedT.σ1(ω) forx=0.011 shows different behaviours in the PI and PM regions. The two curves measured at 300 K highlight the presence of large hysteresis: the curve at 300 K reached from the PI side (on cooling) shows the expected insulating behaviour that is not fully recovered when 300 K is reached from the PM phase (on heating). In the PI phase only a small difference is found inσ1(ω) ofx=0.011 and 0.028. Solid symbols inb–drepresent dc values as measured in ref.7on crystals of the same batch. (c)σ1(ω) in the PM phase highlighting the difference between V2O3and (V0.989Cr0.011)2O3showing a clear Drude peak and a poor metallic behaviour, respectively. (d) Experimental and (e) theoretical reconstruction ofσ1(ω) in the T-induced PM phase, succesfully obtained by modelling, with the sameqandfparameters (see text), the coexistence of metallic and insulating domains through the effective medium approximation (EMA). Figure 1: Temperature-dependent infrared measurements. ( a ) Schematic phase diagram as defined in (ref. 1 ); markers indicate the measurements shown in ( b – e ) in the same colour coding. ( b ) σ 1 ( ω ) of (V 1− x Cr x ) 2 O 3 for x =0.011 and 0.028 at selected T . σ 1 ( ω ) for x =0.011 shows different behaviours in the PI and PM regions. The two curves measured at 300 K highlight the presence of large hysteresis: the curve at 300 K reached from the PI side (on cooling) shows the expected insulating behaviour that is not fully recovered when 300 K is reached from the PM phase (on heating). In the PI phase only a small difference is found in σ 1 ( ω ) of x =0.011 and 0.028. Solid symbols in b – d represent dc values as measured in ref. 7 on crystals of the same batch. ( c ) σ 1 ( ω ) in the PM phase highlighting the difference between V 2 O 3 and (V 0.989 Cr 0.011 ) 2 O 3 showing a clear Drude peak and a poor metallic behaviour, respectively. ( d ) Experimental and ( e ) theoretical reconstruction of σ 1 ( ω ) in the T-induced PM phase, succesfully obtained by modelling, with the same q and f parameters (see text), the coexistence of metallic and insulating domains through the effective medium approximation (EMA). Full size image It was soon evident that this simple scheme hides a more complicated scenario. In their conducting phase weakly Cr-doped samples show a poor metallic behaviour (resistivity ~10 −2 Ω cm) [1] , [2] . Moreover the structure of (V 0.989 Cr 0.011 ) 2 O 3 is described as coexistence of an α-phase, with lattice parameters close to those of metallic V 2 O 3 at 400 K, and a β-phase with basically the same structure as at higher Cr content [3] , [4] . In addition, EXAFS measurements [5] suggest the essential role played by the local lattice strain that occurs in the Cr-doped compounds: Cr contracts the Cr–V bond, inducing a concomitant elongation of the V–V distances [5] . As shown by theoretical calculation based on the local-density approximation combined with dynamical mean field theory (LDA+DMFT) [6] , a longer V–V bond is associated with the PI insulating phase [3] . Besides these open issues concerning the T-induced MIT, further questions are raised by studies under external pressure: in (V 0.989 Cr 0.011 ) 2 O 3 , for instance, a conducting phase is obtained at room temperature if P >3 kbar [7] , and early investigations stated that applying pressure is equivalent to decreasing the Cr content [8] . Recently it was observed that different electronic structures for the metallic phase can be obtained when the PI–PM transition is induced by doping temperature or pressure [9] , challenging the simple scenario of the McWhan phase diagram [1] . In this paper we explore the phase diagram of Cr-doped V 2 O 3 from macroscopic to microscopic scales, by combining three spectroscopies with different lateral resolution, that is infrared (IR), scanning photoemission microscopy (SPEM) and X-ray diffraction (XRD), with LDA+DMFT calculations. We find unambiguous evidence of an electronic phase separation in the T-induced PM phase. The poor metallic behaviour is therefore explained in terms of a coexistence of metallic and insulating domains stabilized by structural defects. Both IR and XRD measurements demonstrate that external pressure can drive the MIT much closer to a genuine Mott transition, leading eventually to a homogeneous metallic phase, as expected insofar in (V 0.989 Cr 0.011 ) 2 O 3 . However, to recover the lattice parameters and the electronic structure of undoped V 2 O 3 a much higher pressure is needed than expected from macroscopic transport measurements [1] , [7] . These findings throw new light on the properties of vanadium sesquioxide. In particular the phase separation occurring along some pathways across the PI–PM transition translates into intrinsically different properties of the corresponding PM phase. Infrared spectroscopy and photoemission scanning microscopy In the PM state at 220 K, the optical conductivity σ 1 ( ω ) of (V 0.989 Cr 0.011 ) 2 O 3 , reported in Figure 1b , shows a pseudogap in the far IR but absolutely no Drude-like contribution. One may also notice that the extrapolation to ω =0 is in excellent agreement with the dc conductivity. The absence of a Drude term is in striking contrast with what is observed in V 2 O 3 at the same temperature ( Fig. 1c ), and implies that within the PM region of the phase diagram the metallic properties can change dramatically. On the contrary, in the PI phase the spectrum of (V 0.989 Cr 0.011 ) 2 O 3 is akin to that of (V 0.972 Cr 0.028 ) 2 O 3 : both spectra are characterized by a small insulating gap associated with an absorption band centred around 3,000 cm −1 . The T-induced PI–PM transition thus corresponds only to a weak redshift of the spectral weight ( Fig. 1b ). The optical data also show a strong thermal hysteresis ( Fig. 1b ): on cooling the MIT occurs below ~260 K; on heating thereafter the sample, the PM phase remains stable up to 275 K and also at 300 K the PI phase is not fully recovered. The absence of a metallic contribution in the optical spectra of the x =0.011 sample calls for further investigations, especially because recent photoemission measurements on crystals from the same batch detected a clear metallic quasiparticle peak [10] , [11] , [12] , [13] , when performed with sufficient bulk sensitivity [14] . To better understand this apparently contradictory results, we performed SPEM with submicrometric spatial resolution [15] , revealing an inhomogeneous electronic distribution in the PM phase. 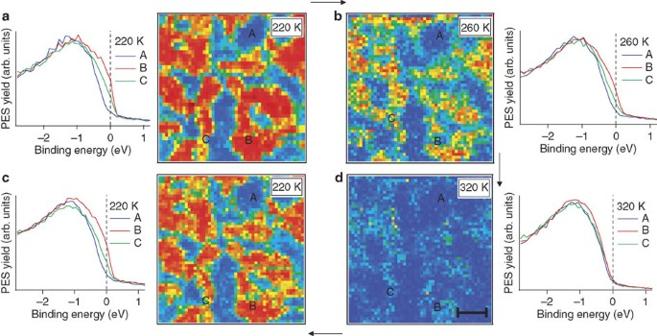Figure 2: Temperature-dependent photoemission microscopy measurements. Scanning photoemission microscopy images and spectra on (V0.989Cr0.011)2O3, collected at 27 eV photon energy and at different temperatures on a 50×50 μm sample area. The images are obtained with standard procedures to remove background and topography effects16. The pictorial contrast between metallic and insulating zones is obtained from the photoemission intensity at the Fermi level17, normalized by the intensity on the V3d band (binding energy −1.2 eV). The lateral variation of this normalized intensity is represented in the colour scale (the intensity scale is the same for all four maps) from its minimum value, in violet, to its maximum, in red, and is therefore a direct visualization in real space of the metallicity of the system. Inhomogeneous properties are found within the PM phase atT=220 K (a) and 260 K (b), where metallic (in red) and insulating (in blue) domains coexist. To recover the PI phase, we heated the sample to 320 K, to make sure that the hysteresis effects still present at 300 K (seeFig. 1) are overcome: at this temperature (c) a homogenous insulating state is obtained. After a whole thermal cycle (d) the metallic regions can be found in the same position and shape as in (a). The photoemission spectra (outer panels) from selected representative areas (A, B, C) corroborate this interpretation. The scale bar in panel c represent 10μm. The maps of the photoelectron yield at E F [16] , [17] are plotted in Figure 2 together with representative photoemission spectra. It should be pointed out that our experimental geometry [15] and photon energy (27 eV) did not allow the collection of sufficiently bulk sensitive photoelectron spectra [10] , [11] , [12] , [13] . Thus the spectra corresponding to the metallic phase do not show a pronounced quasiparticle peak. Nevertheless, the difference between insulating and metallic phases is unambiguous. Consequently, we interpret the photoemission microscopy images as representative of the topmost part of the metallic and insulating domains, whose thickness is expected to be comparable to the IR probing depth. This penetration depth is sufficient to provide the excellent agreement between optical and the dc conductivity obtained with transport measurements. With these maps we resolve metallic and insulating domains that appear as T < T MIT and persist in the PM phase. A uniform insulating behaviour is found instead in the PI phase ( Fig. 2c ), showing that the PM state only is strongly phase separated. Furthermore, when the sample is cooled down again ( Fig. 2d ), the metallic and insulating domains are still found in the same position and with a similar shape, clearly showing that they form around specific points in the sample. It is natural to correlate these nucleation centres to structural inhomogeneites in the material. Such a tendency towards phase separation is related to the correlation energy that fosters a thermodynamic instability in the vicinity of the Mott transition [18] , [19] . This is anologous to the liquid–vapour transition, and we can hence visualize the PI–PM transition as the formation of metallic clouds within an insulating sky. Figure 2: Temperature-dependent photoemission microscopy measurements. Scanning photoemission microscopy images and spectra on (V 0.989 Cr 0.011 ) 2 O 3 , collected at 27 eV photon energy and at different temperatures on a 50×50 μm sample area. The images are obtained with standard procedures to remove background and topography effects [16] . The pictorial contrast between metallic and insulating zones is obtained from the photoemission intensity at the Fermi level [17] , normalized by the intensity on the V3d band (binding energy −1.2 eV). The lateral variation of this normalized intensity is represented in the colour scale (the intensity scale is the same for all four maps) from its minimum value, in violet, to its maximum, in red, and is therefore a direct visualization in real space of the metallicity of the system. Inhomogeneous properties are found within the PM phase at T =220 K ( a ) and 260 K ( b ), where metallic (in red) and insulating (in blue) domains coexist. To recover the PI phase, we heated the sample to 320 K, to make sure that the hysteresis effects still present at 300 K (see Fig. 1 ) are overcome: at this temperature ( c ) a homogenous insulating state is obtained. After a whole thermal cycle ( d ) the metallic regions can be found in the same position and shape as in ( a ). The photoemission spectra (outer panels) from selected representative areas (A, B, C) corroborate this interpretation. The scale bar in panel c represent 10μm. Full size image Although a T-induced structural phase separation was previously proposed on the basis of diffraction [1] , [4] and EXAFS [5] experiments, it was never associated before with an inhomogeneous electronic state. Our data map for the first time the MIT on the microscale, showing metallic and insulating domains that can be naturally linked to the α- and β-lattice structures, respectively. On the basis of these experimental findings in photoemission microscopy, we can also understand the poor metallic behaviour in the PM phase, detected in the optical spectra. To further elaborate on this, we use the effective medium approximation (EMA) [20] that is widely recognized to be meaningful in the presence of microscopic inhomogeneities smaller than the wavelength of the electromagnetic radiation. EMA describes the (complex) dielectric function of an inhomogeneous system [21] , [22] in terms of the optical response of the two components (details in Supplementary Methods ), weighted by the respective volume fraction f and depolarization factor q : Here, and are the complex optical dielectric functions of the metallic and the insulating phase. We reproduce the experimental conductivity in the PM phase of (V 0.989 Cr 0.011 ) 2 O 3 at any T by using as input parameters the α- and β-conductivities as measured in V 2 O 3 [23] and (V 0.972 Cr 0.028 ) 2 O 3 , respectively. In particular previous measurements showed that the optical properties of V 2 O 3 were strongly dependent on lattice modifications [23] . As the lattice parameters of α (V 0.989 Cr 0.011 ) 2 O 3 phase correspond to those of V 2 O 3 at 400 K [1] , [4] , we choose the corresponding 400 K optical conductivity for the EMA reconstruction. Instead, the optical conductivity of (V 0.972 Cr 0.028 ) 2 O 3 , representative of the β-phase, being nearly T independent was chosen at 220 K. Extracting f =0.45±0.05 from the map in Figure 2a (see Supplementary Fig. S1 and discussion in Supplementary Methods ), and leaving q as the only free-fitting parameter, a good agreement between fit (empty squares in Fig. 1d ) and experimental data (solid line) is found for q =0.30±0.05 at 220 K ( q =0.40±0.05 at 300 K), similar to the value found in VO 2 across its first-order MIT [22] . Because f > q the MIT transition is percolative in nature, thus explaining the low dc values measured in samples coming from the same batch. IR measurements associated with SPEM data therefore clarify the poor metallic behaviour observed on a macroscopic spatial scale. DMFT calculations To further support the paramount role played by phase separation for the low-energy excitations of (V 0.989 Cr 0.011 ) 2 O 3 , we compare our IR results with state-of-the-art LDA+DMFT calculations [24] , [25] ( Supplementary Fig. S2 and discussion in Supplementary Methods ). The LDA+DMFT optical conductivity shows a metallic peak in the PM α-phase (yellow line; Fig. 1e) and a gap followed by the t 2g → t 2g excitations in the insulating β-PI phase (grey line; Fig. 1e ). To calculate the LDA+DMFT optical conductivity for the PM phase at x =0.011, we follow what our experimental analysis suggests, namely to take a mixture of the pure α- and β-phases. An important point is that, although EMA in the experimental analysis is (necessarily) performed by assuming the metallic phase to be represented by x =0 and the insulating one by x =0.028, our LDA+DMFT approach allows us to use the 'actual' α- and β-phases at x =0.011 in the EMA formula. Using the same values for the parameters f and q for theory and experiment, we find a LDA+DMFT optical conductivity at x =0.011 (open symbols in Fig. 1e ) that strongly resembles the experimental curve: in particular, its behaviour is markedly insulating-like, as in the experiment. Note that tendencies towards phase separation close to a MIT have been discovered in DMFT before, on the basis of a negative compressibility [18] and a negative curvature of the energy versus volume curve [19] . These tendencies can be further enhanced by the coupling of electronic and lattice degrees of freedom. Pressure-dependent measurements Let us now turn to the P-induced MIT: at the minimum P (1 kbar), σ 1 ( ω ) shows an overall insulating behaviour resembling that at ambient pressure. As P is increased, σ 1 ( ω ) changes abruptly. Indeed, a sudden transfer of spectral weight from above ~3,000 cm −1 to lower frequency builds up a metallic conductivity that well extrapolates to the dc values (solid diamonds in Fig. 3a ), measured on samples of the same batch. The difference from the poor metallic behaviour found in the T-induced PM phase at 220 K (and ambient P) is striking. Nevertheless, even at 15 kbar, the optical conductivity of V 2 O 3 is not yet recovered, challenging the proposed scaling relation between Cr-doping and pressure ( x ~0.011≈ P =4 kbar) obtained by dc resistivity measurements [7] , [8] . The metallicity induced by pressure can be associated with a double process: a weaker phase separation and a modification of the α-domain lattice parameters, which may become more similar to those of pure V 2 O 3 at room temperature. 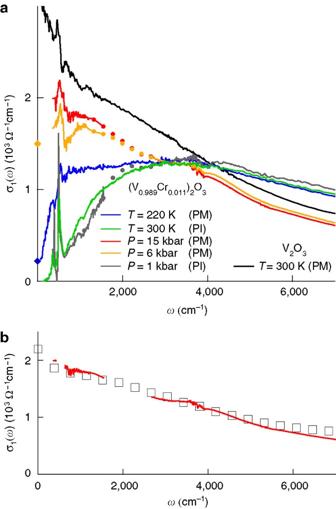Figure 3: Pressure-dependent infrared measurements. (a) Optical conductivity of (V0.989Cr0.011)2O3under pressure (data between 1,600 and 2,700 cm−1, due to the strong diamond phonon absorption, are substituted by markers as a guide for the eye). Under increasing P, the optical conductivity is depleted at energies above 3,000 cm−1and increases below this energy. The curves at 1, 6 and 15 kbar are compared to the PM state of V2O3at 300 K and to the poor metallic phase of (V0.989Cr0.011)2O3at 220 K. In the latter phase no metallic-like increase is built up forω→0, whereas as a function of pressure some coherent transport takes place, as supported also from the resistivity data (solid diamonds inFig. 3a) that allows to extrapolate smoothly the curves toω→0. (b) The experimental reconstruction ofσ1(ω) (red curve same as ina) in the P-induced PM phase obtained by EMA (squares). Figure 3: Pressure-dependent infrared measurements. ( a ) Optical conductivity of (V 0.989 Cr 0.011 ) 2 O 3 under pressure (data between 1,600 and 2,700 cm −1 , due to the strong diamond phonon absorption, are substituted by markers as a guide for the eye). Under increasing P, the optical conductivity is depleted at energies above 3,000 cm −1 and increases below this energy. The curves at 1, 6 and 15 kbar are compared to the PM state of V 2 O 3 at 300 K and to the poor metallic phase of (V 0.989 Cr 0.011 ) 2 O 3 at 220 K. In the latter phase no metallic-like increase is built up for ω →0, whereas as a function of pressure some coherent transport takes place, as supported also from the resistivity data (solid diamonds in Fig. 3a ) that allows to extrapolate smoothly the curves to ω →0. ( b ) The experimental reconstruction of σ 1 ( ω ) (red curve same as in a ) in the P-induced PM phase obtained by EMA (squares). 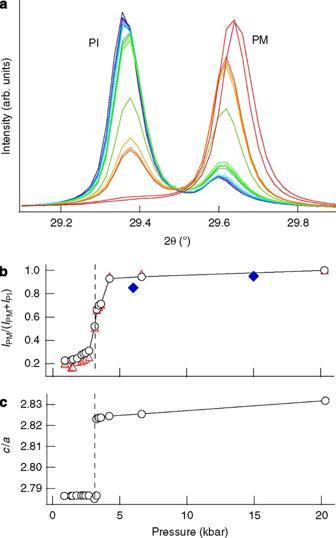Figure 4: Pressure dependent Bragg X-ray diffraction measurements. (a) Bragg X-ray diffraction (300) line of (V0.989Cr0.011)2O3under pressure at room temperature. The peak at the left corresponds to the lattice parameters of the PI phase, whereas the one at the right corresponds to PM. The spectra from violet to red were taken at pressures from 0 to 20 kbar, corresponding to the data points inFigure 4b and c. (b) PM intensity over the total one (PM+PI) as a function ofPfor the (300) line (circles) and for the (214) line (triangles). Solid symbols represent the same quantity calculated from thefEMA parameter (see above). (c)c/aratio of the lattice parameters versusPextracted fromFigure 4a. Full size image To clarify these issues, high-pressure XRD measurements have been performed in the same pressure range and the results for the (300) Bragg line (confirmed also by the similar behaviour on other Bragg peaks) are shown in Figure 4a . Two Bragg peaks appear within a range of ~1 kbar across the MIT, showing that the PI phase coexists with the PM one only in this limited pressure range. A further increase of P strongly reduces the phase separation (see Fig. 4b ), and above 10 kbar the Bragg signal is made almost entirely by the PM component. Figure 4: Pressure dependent Bragg X-ray diffraction measurements. ( a ) Bragg X-ray diffraction (300) line of (V 0.989 Cr 0.011 ) 2 O 3 under pressure at room temperature. The peak at the left corresponds to the lattice parameters of the PI phase, whereas the one at the right corresponds to PM. The spectra from violet to red were taken at pressures from 0 to 20 kbar, corresponding to the data points in Figure 4b and c . ( b ) PM intensity over the total one (PM+PI) as a function of P for the (300) line (circles) and for the (214) line (triangles). Solid symbols represent the same quantity calculated from the f EMA parameter (see above). ( c ) c / a ratio of the lattice parameters versus P extracted from Figure 4a . Full size image These data indicate that a more homogenous electronic state develops in the P-induced PM phase. Indeed, an EMA calculation reproduces the P-dependent optical conductivity (see Fig. 3b ), through the same input curves as before. For the same value of q =0.4 obtained at ambient P and room T, a metallic volume fraction f =0.85 at 6 kbar and 0.95 at 15 kbar can be found. These values (solid symbols in Fig. 4b ) are in good agreement with values obtained from XRD measurements, but much larger than the metallic fraction f =0.45 found at 220 K in the T-induced PM phase through SPEM. Eventually, a metallic volume fraction f ~1 is found at pressures where the c / a value in Figure 4c nearly attains that of pure V 2 O 3 ( c / a ~2.83), thus suggesting the importance of the lattice in the physical properties of V 2 O 3 [23] , [26] . We explored the phase diagram of (V 0.989 Cr 0.011 ) 2 O 3 with a combination of different experimental methods and conjoined LDA+DMFT calculations, with particular attention to the PI–PM transition that can be obtained by changing doping, temperature or pressure. Our results throw new light on the different metallicity of the PM phase obtained by lowering T with respect to the one obtained by applying an external P. We showed that a key role to explain this difference is played by phase separation: in particular, the coexistence of metallic and insulating domains was unambiguously demonstrated in the T-induced PM phase. After a thermal cycle these domains reappear in the same positions and with a similar shape: this memory effect may be related to nucleation centres, with electronic correlations further fostering phase separation. The PM phase reached under pressure is instead much more homogeneous and, by increasing P, it soon covers a raising fraction of the volume. However, it is intrinsically different from pure V 2 O 3 if one compares points that are nominally equivalent in the McWhan phase diagram, as shown by the different lattice parameters. This suggests that, during the phase transition induced by P, the strain between the different lattice parameters between PM and PI seems to be accomodated in a more homogeneous way by reducing their difference. In the T-induced transition, instead, this difference is unchanged and the strain is accomodated inhomogeneously inducing domains with different lattice and electronic properties. Our IR results, obtained by changing doping, temperature and pressure, were captured correctly by using the EMA. Thus, optical conductivity bridges between local probes like photoemission and XRD, which can directly detect the microscopic details of the phase separation, and transport measurements, which are instead sensitive to the occurance of a long-scale metallic property. Thanks to this combination of different methods with intrinsically different spatial scale sensitivity, we were able to clarify the properties of the phase diagram of vanadium sesquioxide from macroscopic to microscopic spatial scales, showing that the phase separation occuring along the different pathways across the PI–PM transition translates into different properties of the PM phase. In conclusion, our investigation shows that the phase diagram of V 2 O 3 , celebrated for its essential simplicity, reveals on a microscopic scale a much richer phenomenology that has to be taken into account in the physical description of this model system. Materials All the measurements on (V 0.989 Cr 0.011 ) 2 O 3 , using different experimental techniques as detailed in this article, were performed on single crystals from the same batch grown at Purdue University. The specimens were thoroughly characterized before the experiments by means of transport measurements (P. Metcalf, private communication), and precisely oriented with XRD. Infrared measurements The temperature-dependent reflectivity ( R ) measurements have been performed at near-normal incidence with the electrical field polarized within the ab plane and by using as a reference a metallic film (gold or aluminium depending on the spectral range) evaporated in situ over the sample surface. A standard low-frequency extrapolation was performed by using a Drude–Lorentz fitting of the measured R by taking into account the dc values of the resistivity measured on samples of the same batch, whereas the high-frequency tail from (ref. 23 ) was merged to the data, to perform reliable Kramers–Kronig transformations. A diamond anvil cell equipped with type IIa diamonds was used to perform pressure-dependent measurements. A hole of about 300 μm diameter was drilled in a 50 μm thick Al gasket, allowing us to span over the desired pressure range (0–15 kbar) in a reproducible and cyclic way. A small piece was cut from the sample measured as a function of T and placed in the sample chamber together with a KBr pellet (used as hydrostatic medium) and the electric field of the radiation was polarized within the ab plane. We took great care of creating a clean sample diamond interface. The pressure was measured in situ with the standard ruby fluorescence technique [27] . To reduce the experimental error of such data, a ruby microsphere was placed inside the sample chamber whereas a second one was placed on the external face of the diamond. Measurements were performed on both ruby balls several times for each pressure, taking therefore in account any slight change in the temperature or in the spectrometer calibration. The incident and reflected light were focused and collected with a cassegrain-based optical microscope equipped with a MCT detector and a bolometer and coupled to a Michelson interferometer. This allowed us to explore the 350–12,000 cm −1 spectral range exploiting the high brilliance of synchrotron radiation at SISSI beamline at ELETTRA storage ring [28] . The measurement procedure was the same as described in refs. 29 , 30 . The conductivity, , has been calculated through Kramers–Kronig transformations, taking into account the diamond-sample interface [31] , [32] , [33] . Data are not shown in the 1,600–2,700 cm −1 due to the strong phonon absorption of diamonds. Photoemission microscopy The photoemission microscopy results were obtained on the spectromicroscopy beamline [15] at the Elettra. Photons at 27 eV were focused through a Schwarzschild objective, to obtain a submicron size spot. The measurements were performed in ultra-high vacuum ( P <2×10 −10 mbar) on in situ prepared surfaces of (V 0.989 Cr 0.011 ) 2 O 3 . Photoelectrons were collected at an emission angle of 65° from the normal, which makes the photoemission spectra and images surface sensitive. A standard photoemission microscopy procedure was used to remove topographic features [34] from the images presented in Figure 2 , and to obtain an unambiguous contrast between metallic and insulating regions [16] : the spectral intensity at the Fermi level E F —high in the PM and absent in the PI phase [11] , [12] —was divided by the intensity recorded at the V3d band. Because the latter remains essentially constant between the PI and PM phases, two-dimentional maps of this ratio give a genuine representation of the lateral variation of metallic and insulating domains. X-ray diffraction The XRD measurements were performed using 17 keV photons dispersed by the CRISTAL beamline at the SOLEIL synchrotron radiation source [35] . Pressure was applied to a (V 0.989 Cr 0.011 ) 2 O 3 powder by means of a membrane-driven diamond anvil cell, and its value in the cell was carefully measured during the measurement sequence using the standard ruby fluorescence method. The transmission of the diamond cell at the photon energy used during these experiments was sufficient to allow a high resolution detection of the main Bragg reflections like the (300) and (214) presented here. How to cite this article: Lupi, S. et al . A microscopic view on the Mott transition in chromium-doped V 2 O 3 . Nat. Commun. 1:105 doi: 10.1038/ncomms1109 (2010).